Imaging enzyme-triggered self-assembly of small molecules inside live cells Self-assembly of small molecules in water to form nanofibres, besides generating sophisticated biomaterials, promises a simple system inside cells for regulating cellular processes. But lack of a convenient approach for studying the self-assembly of small molecules inside cells hinders the development of such systems. Here we report a method to image enzyme-triggered self-assembly of small molecules inside live cells. After linking a fluorophore to a self-assembly motif to make a precursor, we confirmed by 31 P NMR and rheology that enzyme-triggered conversion of the precursor to a hydrogelator results in the formation of a hydrogel via self-assembly. The imaging contrast conferred by the nanofibres of the hydrogelators allowed the evaluation of intracellular self-assembly, the dynamics and the localization of the nanofibres of the hydrogelators in live cells. This approach explores supramolecular chemistry inside cells and may lead to new insights, processes or materials at the interface of chemistry and biology. Driven by supramolecular interactions, for example, hydrophobic interactions and hydrogen bonding, certain small molecules self-assemble in aqueous solution to form nanofibres (or other nanostructures) and consequently result in hydrogels [1] , [2] , [3] , [4] , [5] . Because of their inherent advantages, such as biocompatibility, biodegradability and morphological resemblance of extracellular matrix, supramolecular nanofibres/hydrogels promise applications in cell culture, drug delivery and tissue engineering, and recently have attracted increased interests in the development of new biomaterials [6] , [7] , [8] , [9] , [10] , [11] , [12] , [13] . Besides the incorporation of epitopes or bioactive molecules in the hydrogelators [6] , [14] , [15] , it is also important to evaluate the distribution of the nanofibres of the hydrogelators in both extracellular and intracellular environment, and to understand their interactions with cellular components. Although it is relatively straightforward to introduce a fluorophore into a hydrogelator [16] for imaging the location of hydrogelators in a biological setting, it is rather difficult to distinguish individual fluorescent hydrogelators and the corresponding nanofibres because of the little difference between the two cases. In fact, owing to the limited exploration on fluorescent hydrogelators and hydrogels [17] , there is no known molecule that only exhibits fluorescence after the self-assembly to form the nanofibres. To solve the above dilemma, we chose to design, synthesize and characterize a new precursor of fluorescent hydrogelator for evaluating the nanofibres of the hydrogelators inside cells. We expect the precursor and the individual hydrogelators to exhibit low fluorescence, and the nanofibres of the hydrogelators to display bright fluorescence. We use enzymatic hydrogelation [18] , [19] —an enzymatic reaction to convert the precursor to the hydrogelator for forming the nanofibres/hydrogels—to produce the nanofibres in cells for several reasons. First, there is a drastic difference between extracellular and intracellular environments in enzyme distributions, which offers a reliable contrast for imaging. Second, compared with the change of pH, temperature or ionic strength, enzymatic reaction is a biocompatible strategy that works in both extra- and intracellular environments [20] , [21] , [22] , [23] , [24] , [25] , [26] , [27] . Third, in enzymatic hydrogelation, while the precursors diffuse freely, the formation of the nanofibres of the hydrogelators, as a convergent process, reduces the diffusion of the hydrogelators. Fourth, enzymatic hydrogelation also provides a new way to reveal the spatiotemporal files of specific enzymes, which may help understand the interaction of the nanofibres with cellular components. By designing and generating a precursor NapFFK(NBD)Yp ( 2 ) of fluorescent hydrogelator ( 3 ), we not only determined that endoplasmic reticulum (ER) is the location of the self-assembled fluorescent hydrogelators inside live cells, but also observed the growth of the nanofibres from ER towards the edge of the cells. These results, obtained from imaging enzyme-triggered self-assembly of small molecules inside live cells, illustrates a novel approach for studying the self-assembly of small molecules inside cells, a potentially important, yet unexplored, subject at the interface of supramolecular chemistry and biology [28] . 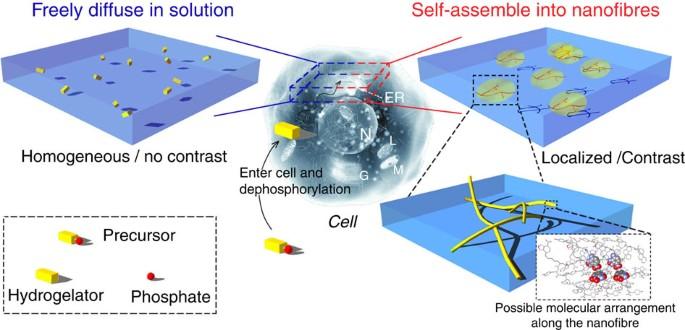Figure 1: Principle of imaging enzyme-triggered supramolecular self-assembly inside cells. After an enzymatic conversion inside the cell, the precursor turns to the corresponding hydrogelator, a more hydrophobic molecule that self-assembles to form nanofibres at certain concentration. When the precursors are outside cells or the concentration of hydrogelator is too low to form nanofibres, those precursors or hydrogelators diffuse freely, distribute homogeneously, fluoresce identically within each pixel and thus show little contrast. Once the concentration of hydrogelator reaches high enough to form nanofibres, these nanofibres have more fluorophores within each pixel than the rest solution, and the fluorophores (as shown in CPK model) within nanofibres are localized, therefore the nanofibres fluoresce more brightly and generate the contrast. ER, endoplasmic reticulum; G, Golgi apparatus; L, lysosome; M, mitochondria; N, nucleus. Principle for imaging molecular self-assembly inside cells Figure 1 shows the principle of the fluorescent imaging of this enzyme-triggered self-assembly process inside cells. Being observed at the focal plane of the microscope, the precursor of the hydrogelator, bearing a fluorophore and an enzyme trigger (for example, a tyrosine phosphate residue as the substrate of alkaline phosphatase (ALP)), dissolves well in water and diffuses freely to result in the homogeneous distribution of the fluorophores. Being excited, the precursors in solution emit identically in each pixel within the optical thickness of the focal plane, thus affords little contrast for imaging. In the presence of the enzyme, the precursors turn into the hydrogelators, which, at above certain concentration, self-assemble to form nanofibres and to be localized. Obviously, many hydrogelators in the nanofibres lead to the high density of fluorophores in the nanofibres, which contribute much higher fluorescence to some pixels than the rest of solution does, thus affording the excellent contrast for imaging. Overall, the condensation and localization of the fluorophores render the nanofibres themselves to be distinctly visible in fluorescent microscopy [29] , [30] , [31] . Figure 1: Principle of imaging enzyme-triggered supramolecular self-assembly inside cells. After an enzymatic conversion inside the cell, the precursor turns to the corresponding hydrogelator, a more hydrophobic molecule that self-assembles to form nanofibres at certain concentration. When the precursors are outside cells or the concentration of hydrogelator is too low to form nanofibres, those precursors or hydrogelators diffuse freely, distribute homogeneously, fluoresce identically within each pixel and thus show little contrast. Once the concentration of hydrogelator reaches high enough to form nanofibres, these nanofibres have more fluorophores within each pixel than the rest solution, and the fluorophores (as shown in CPK model) within nanofibres are localized, therefore the nanofibres fluoresce more brightly and generate the contrast. ER, endoplasmic reticulum; G, Golgi apparatus; L, lysosome; M, mitochondria; N, nucleus. Full size image Design and synthesis of the precursor Based on the principle illustrated in Fig. 1 , we first designed and synthesized the precursor. 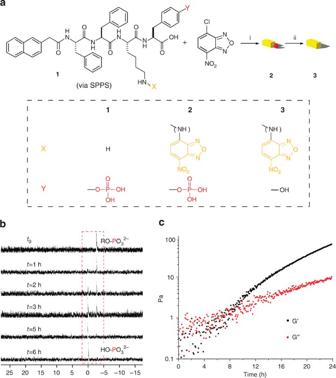Figure 2: Molecular transformation during the enzymatic hydrogelation process. (a) The synthesis route of the precursor2and the generation of the fluorescent hydrogelator3via an enzyme-catalysed dephosphorylation. (i) Na2CO3, methanol, water, 50 °C, 2 h; (ii) ALP. (b,c) The dephosphorylation and hydrogelation process of the solution of2(pH 7.4, 0.6 wt%, 5.92 mM) after being mixed with ALP (20 U ml−1): (b)31P NMR to show enzymatic dephosphorylation (that is, decrease of the phosphorous ester peak and increase of phosphate peak) and (c) rheometry to show the progress of the hydrogelation of3that is converted from2(that is, at the gel state, storage modulus (G′) dominates loss modulus (G′′)). Figure 2 shows the design of the precursor 2 , a combination of a fluorophore, 4-nitro-2,1,3-benzoxadiazole (NBD), and a phosphorous ester on the tyrosine residue of a small peptide ( 1 ). The NBD group is a fluorophore known to give more intense fluorescence in hydrophobic environment than in water and has found applications in the imaging of self-assembly of tubulins [32] . Thus, the use of NBD warrants a high quantum yield of the fluorophore inside the nanofibres. The dephosphorylation of 2 catalysed by an ALP affords the corresponding hydrogelator 3 , which, as a more hydrophobic molecule than the precursor, is able to self-assemble in water to form nanofibres and to result in the hydrogel. While the tetrapeptidic backbone of 3 provides the basis for intermolecular hydrogen bonding, the naphthyl group and phenyl groups (on phenylalanine) favour intermolecular aromatic–aromatic interactions. These intermolecular interactions (for example, hydrogen bonding and hydrophobic interactions) facilitate the self-assembly and the formation of the nanofibres and the hydrogel of 3 . According to the molecular design, the synthetic process of 2 is rather straightforward. After the synthesis of the peptidic motif NapFFKYp ( 1 ) via solid phase peptide synthesis through an effective Fmoc-strategy [33] , we labelled 1 with the amine-reactive fluorogenic reagent (7-chloro-4-nitro-2,1,3-benzoxadiazole (NBD-Cl)) and obtained the precursor 2 in 67% yield ( Fig. 2a ). Figure 2: Molecular transformation during the enzymatic hydrogelation process. ( a ) The synthesis route of the precursor 2 and the generation of the fluorescent hydrogelator 3 via an enzyme-catalysed dephosphorylation. (i) Na 2 CO 3 , methanol, water, 50 °C, 2 h; (ii) ALP. ( b , c ) The dephosphorylation and hydrogelation process of the solution of 2 (pH 7.4, 0.6 wt%, 5.92 mM) after being mixed with ALP (20 U ml −1 ): ( b ) 31 P NMR to show enzymatic dephosphorylation (that is, decrease of the phosphorous ester peak and increase of phosphate peak) and ( c ) rheometry to show the progress of the hydrogelation of 3 that is converted from 2 (that is, at the gel state, storage modulus (G′) dominates loss modulus (G′′)). Full size image Self-assembly of fluorescent hydrogelators in vitro After obtaining 2 , we established enzyme-triggered self-assembly of fluorescent hydrogelators in vitro . We used 31 P NMR to examine the rate of dephosphorylation of 2 and applied rheometry to determine the hydrogelation point of 3 . In the 31 P NMR experiment, we monitored the enzymatic dephosphorylation hourly with an acquisition time of 3 min 27 s (256 repetitions). As shown in Fig. 2b , the 31 P peak of the phosphorous ester almost completely disappears 6 h after the addition of the enzyme, suggesting the full conversion of 2 to 3 . The rheological test ( Fig. 2c ) shows that the hydrogelation point emerges 8 h after the addition of the enzyme, indicating that the hydrogelation occurs after the completion of the enzymatic dephosphorylation. The visual observation and the transmission electron micrograph (TEM) of the hydrogel agree with the process of the dephosphorylation confirmed by 31 P NMR and rheology. At pH 7.4 and the concentration of 0.6 wt%, 2 forms a transparent solution ( Fig. 3a , left), but exhibits little fluorescence ( Supplementary Fig. S1A and B ). At 4 h after the addition of ALP (20 U ml −1 ), the solution still shows little fluorescence. The mixture finally becomes a transparent and fluorescent hydrogel ( Fig. 3a , right and Supplementary Fig. S1C and D ) 8 h after the addition of the enzyme. Negative-staining TEM [34] of the hydrogel of 3 reveals that the self-assembled nanofibres with quite uniform diameters (10±2 nm) entangle with each other to form a network as the matrices of the hydrogel ( Fig. 3b ). These results not only show that 3 self-assemble to form nanofibres but also indicate that the formation of nanofibres (or hydrogelation) enhances the fluorescent signal of NBD. 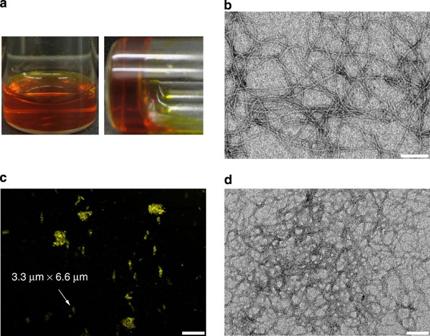Figure 3: Enzyme-triggered self-assembly at different concentrationsin vitro. (a) Optical images of (left) the solution of2(0.6 wt%, pH 7.4) and (right) the hydrogel of3by treating2(0.6 wt%) with ALP (20 U ml−1) at pH 7.4. (b) The TEM image of the negatively stained nanofibres in the hydrogel of3. (c) The confocal fluorescent microscope image (×63 oil objective lens) shows the appearance of bright spots in the solution of2(500 μM, pH 7.4 in PBS buffer) with the treatment of ALP (20 U ml−1). (d) TEM image shows that a fluorescent spot shown in (c) consists of the network of nanofibres. (Scale bar,b, 100 nm;c, 25 μm;d, 100 nm.) Figure 3: Enzyme-triggered self-assembly at different concentrations in vitro . ( a ) Optical images of (left) the solution of 2 (0.6 wt%, pH 7.4) and (right) the hydrogel of 3 by treating 2 (0.6 wt%) with ALP (20 U ml −1 ) at pH 7.4. ( b ) The TEM image of the negatively stained nanofibres in the hydrogel of 3 . ( c ) The confocal fluorescent microscope image (×63 oil objective lens) shows the appearance of bright spots in the solution of 2 (500 μM, pH 7.4 in PBS buffer) with the treatment of ALP (20 U ml −1 ). ( d ) TEM image shows that a fluorescent spot shown in ( c ) consists of the network of nanofibres. (Scale bar, b , 100 nm; c , 25 μm; d , 100 nm.) Full size image The enhanced fluorescence of NBD in the hydrogel arises from the higher quantum yield of NBD in a hydrophobic environment [35] . According to the fluorescent spectra of the solution of 2 ( Supplementary Fig. S2 ), the fluorescence of 2 decreases with the increase of its concentration, suggesting that the self-quenching likely originates from the increase of the concentration of 2 . At the concentration of 0.6 wt% (5.92 mM) in an aqueous solution, the fluorophore NBD fluoresces little because of the hydrophilic environment and self-quench phenomenon. During the transition from solution to hydrogel, hydrogelators of 3 self-assemble to form nanofibres. Along either the longitudinal direction or axial direction, the dimensions of these nanofibres are larger than the two layers of 3 ; thus, many molecules of 3 must embed inside the nanofibres that provide a hydrophobic microenvironment ( Supplementary Fig. S3 ), which allows NBD to fluoresce with a higher quantum yield than in aqueous solution. In addition, the formation of the nanofibres also reduces the diffusion-originated non-irradiative decay. Therefore, the overall effect is that the hydrogel of 3 exhibits fluorescence despite that self-quenching also occurs in the nanofibres of 3 ( Supplementary Fig. S4 ). This result validates the choice of NBD as the fluorophore of the hydrogelators. Although the hydrogelation is, probably, the easiest way to identify molecular self-assembly in water, the self-assembly to form the nanofibres could occur without the formation of a bulk hydrogel. Thus, the fluorescence associated with the nanofibres of 3 may serve as a useful and more sensitive assay than hydrogelation for reporting the formation of the nanofibres via self-assembly. To verify whether this assumption is valid, we examined the enzyme-triggered self-assembly of the fluorescent hydrogelators below the critical gelation concentration (cgc) in vitro. After the addition of ALP (20 U ml −1 ) into the solution of 2 (500 μM, in PBS buffer) in which the concentration is below the cgc (2.0 mM, Supplementary Fig. S5 ) required for the hydrogelation of 3 , we found a significant amount of highly fluorescent micron-size regions under confocal fluorescent microscope ( Fig. 3c ). As noticed, these spots hardly move and remain in the solution of 3 . These spots exhibit excellent contrast to the background, suggesting that they are composed of localized and concentrated 3 . While TEM of the negative-stain solution of 2 at 500 μM shows no aggregates ( Supplementary Fig. S6 ), the TEM of the above sample of 3 reveals that these regions contain nanofibres with the length of several microns and the width of 8±2 nm as shown in Fig. 3d ( Supplementary Fig. S7 for the full scope of the spots). The dimensions of the nanofibre networks are similar to the sizes of the spots shown in Fig. 3c . Thus, the observed fluorescence serves as the indication for the formation of the nanofibres formed by the self-assembly of 3 . In addition, the static light scattering of the solution of 2 exhibits little scattering, but the signal of scattering increases dramatically after the addition of ALP. This result ( Supplementary Fig. S8 ) agrees with the observation from TEM and fluorescence. Self-assembly of fluorescent hydrogelators in live cells As the self-assembly of 3 results in nanofibres that fluoresce much brighter than the rest of unassociated molecules of 2 or 3 , 2 is a valid candidate for studying molecular self-assembly of small molecules in cells. The in vitro test described above, which shows that 500 μM of 3 affords self-assembled nanofibres network, suggests that 500 μM of 3 is sufficient for intracellular formation of nanofibres. In addition, our previous results show that the minimum concentration required for intracellular hydrogelation of a similar compound is around 1/4 of the cgc of the hydrogelator in the buffer (without cells) [24] . Moreover, the cell viability test shows that 2 has little cytotoxicity to HeLa cells even at 500 μM and over the period of 3 days ( Supplementary Fig. S9 ), indicating that 2 and 3 are suitable candidates for the construction of nanomaterials inside cells for further exploration. So, we incubated HeLa cells with 2 at two concentrations: 500 μM and 50 μM. As the latter is far below the minimum concentration for hydrogelation in cells, it serves as the negative control of the formation of nanofibres and the hydrogelation. While the concentration of 2 barely changes outside the cells, 2 turns into 3 continuously inside cells, which reaches a non-equilibrium steady state. Because of the variation of the copy numbers of phosphatases in cells, it is impossible to synchronize the enzymatic conversion. Therefore, we observed the dynamics of 3 inside a single live cell in real time by recording the fluorescent images of these live cells at different time points after the addition of 2 to the cell culture ( Fig. 4 ; Supplementary Movie 1 ). 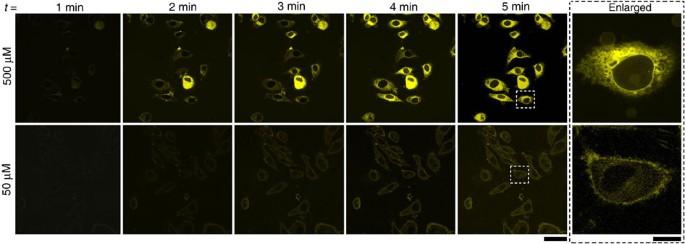Figure 4: Enzyme-trigged self-assembly inside live cells. Fluorescent confocal microscope images show the time course of fluorescence emission inside the HeLa cells incubated with 500 or 50 μM of2in PBS buffer, which shows the different distribution of fluorophores inside living cells. Scale bar, 50 μm for time course panels and 10 μm for the enlarged panels. Figure 4: Enzyme-trigged self-assembly inside live cells. Fluorescent confocal microscope images show the time course of fluorescence emission inside the HeLa cells incubated with 500 or 50 μM of 2 in PBS buffer, which shows the different distribution of fluorophores inside living cells. Scale bar, 50 μm for time course panels and 10 μm for the enlarged panels. Full size image Fluorescent imaging shows the accumulation of fluorophores at different rates and characteristics at those two concentrations (500 and 50 μM). After the addition of 500 μM of 2 to the cells, the emission of 2 outside cells remains dim during the whole experiment, which provides a clear background and enables the real-time visualization of the development of fluorescence inside live cells. The cells incubated with 2 become slightly fluorescent within 80 s, and a bright fluorescent area appears near the nucleus in one of the cells after 3 min. After 5 min, all the cells glow brighter at the centre of the cytoplasm than around the outer membrane of the cells. This localized fluorescence not only indicates the formation of the nanofibres/hydrogels inside live cells (which is much faster than in vitro experiment) but also qualitatively suggests that the total phosphatase activity is much higher inside live cells than the concentration (20 U ml −1 ) used in the in vitro experiment. On the other hand, in the cells treated with 50 μM of 2 , the fluorescence emission intensity changes little inside cells; instead the membrane is slightly brighter than the cytoplasm, which is normal and mainly owing to the membrane at the orthogonal to the image plane [30] . If the fluorescence of NBD at 500-μM incubation concentration of 2 were owing to the binding of 2 or 3 to hydrophobic pockets somewhere in the cell, we would observe strong fluorescence when the cell was incubated at 50 μM of 2 . The lack of strong fluorescence inside the cell at 50 μM of 2 excludes the possibility that the observed fluorescence, at 500 μM of 2, originates from nonspecific binding to hydrophobic pockets of intracellular biomembranes or only dephosphorylation. The most notable observation in the case of 500 μM of 2 is that the increase of the brightest fluorescent area centres inside the cytoplasm and the fluorescence emerges from the centre of the cytoplasm towards the edge of the cells, a direction opposite to the diffusion of 2 into the cells. As the fluorescence increases against the concentration gradient of 2 and the in vitro test proves that the self-assembly of 3 results in the fluorescence, the bright fluorescence suggests the self-assembly of 3 at the centre of the cytoplasm. Moreover, because the formation of 3 requires the dephosphorylation of 2 catalysed by phosphatases, the bright spots also reveal the distribution of phosphatases inside cells. Self-assembly of 3 is concentration dependent and occurs around sub-mM for a significant formation of molecular aggregate. As the concentration at this range would cause most of the organic dyes to self-quench, we have identified that the optimal concentration of 3 for cellular application is 500 μM based on fluorescence spectrum study of a serial dilution of 2 and 3 . This result suggests that care should be paid to find out optimized conditions/concentration for cellular applications. Self-assembly originates from the ER It is also worth to mention that although the self-assembly of 3 initiates sporadically among these cells, the spatial profiles are quite similar, that is, nearby the nucleus and in the region of ER. Thus, most of the self-assembly of 3 occurs at the ER. This presumption is consistent with the cell fraction experiment ( Fig. 5a ), which shows that the ER-containing cell fraction triggers the fastest hydrogelation ( Fig. 5b ) among the cell fractions [36] . In another experiment, we incubated the HeLa cells with 2 (500 μM) for 1 h before subjecting the cell to fractionation. The TEM images of the fractions N , M and P of the treated cell show substantial amount of nanofibres, suggesting the formation of the nanofibres inside cells ( Fig. 6 ). Although the TEM of fraction N shows the nanofibres of 3 , the image in Fig. 4 excludes the possibility that the nanofibres of 3 exist in the nucleus. As the formation of the nanofibres of 3 is protein tyrosine phosphatase (PTP1B)-dependent and there is no report of PTP1B in the mitochondria of HeLa cells, it is unlikely that the nanofibres of 3 form inside mitochondria. Thus, the observation of the nanofibres in fractions N and M likely originates from the high molecular weight of the nanofibres of 3 that makes them more prone to sedimentation. Moreover, the observed nanofibres unlikely are microtubules because no similar nanofibre exists in the control (that is, HeLa cells without incubating with 2 ). 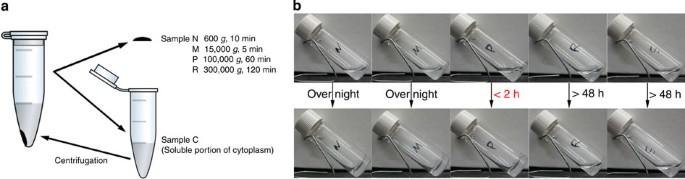Figure 5: Cell fractionation and gelation experiments. (a) The cell fragmentation procedure36to separate pellet sample. N, Nuclei; pellet sample M, mitochondria, lysosomes, peroxisomes; pellet sample P, plasma membrane, microsomal fraction (fragments of ER), large polyribsomes; pellet sample R, ribosomal subunits, small polyribosomes; supernatant sample C, soluble portion of cytoplasm (Cytosol). Pellets N, M, P and R were all redispersed in 200 μl of PBS for further test. (b) Optical images show the hydrogelation speed of each sample by mixing 100 μl of each diluted cell fraction and 200 μl of 9 mg ml−1of1dissolved in PBS. Cell fraction P can induce the hydrogelation much faster (within 2 h) than fractions N and M (overnight) while fractions R and C do not lead to a stable hydrogel. Figure 5: Cell fractionation and gelation experiments. ( a ) The cell fragmentation procedure [36] to separate pellet sample. N, Nuclei; pellet sample M, mitochondria, lysosomes, peroxisomes; pellet sample P, plasma membrane, microsomal fraction (fragments of ER), large polyribsomes; pellet sample R, ribosomal subunits, small polyribosomes; supernatant sample C, soluble portion of cytoplasm (Cytosol). Pellets N, M, P and R were all redispersed in 200 μl of PBS for further test. ( b ) Optical images show the hydrogelation speed of each sample by mixing 100 μl of each diluted cell fraction and 200 μl of 9 mg ml −1 of 1 dissolved in PBS. Cell fraction P can induce the hydrogelation much faster (within 2 h) than fractions N and M (overnight) while fractions R and C do not lead to a stable hydrogel. 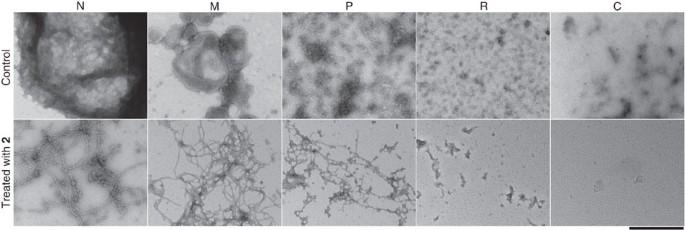Figure 6: TEM images of the cell fractions before and after enzyme-trigged formation of the molecular nanofibres. According to the standard protocol36, HeLa cells were fractioned and divided into five parts, named N, M, P, R and C. The first row shows the typical morphology from each fraction of HeLa cells. The second row shows the typical morphology from each fraction of HeLa cells that were preincubated with2(500 μM) for 1 h. Scale bar, 500 nm. Full size image Figure 6: TEM images of the cell fractions before and after enzyme-trigged formation of the molecular nanofibres. According to the standard protocol [36] , HeLa cells were fractioned and divided into five parts, named N, M, P, R and C. The first row shows the typical morphology from each fraction of HeLa cells. The second row shows the typical morphology from each fraction of HeLa cells that were preincubated with 2 (500 μM) for 1 h. Scale bar, 500 nm. Full size image As PTP1B is a phosphatase known to localize at the cytoplasmic face of the ER [37] , we used an inhibitor of PTP1B (CinnGEL 2Me, 25 μM) to co-incubate with the HeLa cells and the precursor ( 2 ). We observed the delay of the fluorescence ( Fig. 7 ). For example, at 7.5 min, there is no fluorescent cell when the PTP1B inhibitor presents in the medium. After 1-h incubation, 70% cells are fluorescent without the co-incubation of the PTP1B inhibitor, but only 21% cells are fluorescent in the presence of the PTP1B inhibitor. This result confirms that PTP1B is the major phosphatase that catalyses the dephosphorylation of 2 to result in the formation of the nanofibres of 3 in the ER. The rate difference for the in vivo experiment and the in vitro (that is, 31 P NMR) experiment may arise from the concentration and activity difference of the phosphatases in vivo and in vitro . The activity of ALP purchased (Biomatic Co., A1130) has a activity of 3,000 U mg −1 ; the PTP 1B localized at ER and has an activity of 46,780 U mg −1 (soluble fractions) or 42,710 U mg −1 (particulate fractions) [38] (1 unit=release of 1 nmol phosphate per minute). As the activity of PTP1B is about 15 times higher than that of ALP, it is reasonable that the dephosphorylation of 2 inside cells occurs one order of magnitude faster than in vitro . 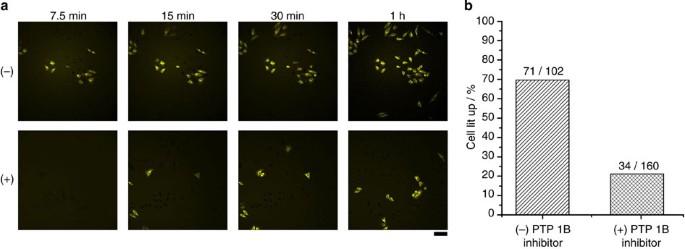Figure 7: PTP1B-dependent self-assembly inside live cells. (a) Time sequences of the HeLa cells treated with 500 μM of2without (−) or with (+) the PTP1B inhibitor (25 μM) (scale bar, 100 μm); (b) The cell count shows the difference of the percentage of fluorescent cells without and with the PTP1B inhibitor at the point of 1 h after the addition of 500 μM of2; 71/102 means 71 cells are fluorescent in the total of 102 cells. Figure 7: PTP1B-dependent self-assembly inside live cells. ( a ) Time sequences of the HeLa cells treated with 500 μM of 2 without (−) or with (+) the PTP1B inhibitor (25 μM) (scale bar, 100 μm); ( b ) The cell count shows the difference of the percentage of fluorescent cells without and with the PTP1B inhibitor at the point of 1 h after the addition of 500 μM of 2 ; 71/102 means 71 cells are fluorescent in the total of 102 cells. Full size image This work, as the first example that combines fluorescence, enzymatic reactions and self-assembly, provides a minimum model structure for studying the self-assembly of small molecules inside cells, which involves cellular processes to construct the designed nanostructures in situ . Though it is unable to determine the location of the nanofibres in the cells, the fractionation experiment unambiguously confirms the formation of the nanofibres inside the cells. By inhibiting the phosphatase (that is, PTP1B) with a known cellular location (that is, ER), we are able to infer the location of the nanofibres. Therefore, this work demonstrates the construction of nanostructures via enzyme-triggered supramolecular self-assembly inside live cells without forming the covalent bond. This approach could be applied to self-assembly triggered by other enzymes when the distribution of the enzymes is well defined. In addition, the resulted molecular nanostructure bears the intrinsic advantages of reversibility and biodegradability, which fundamentally differs from the result reported by Rao and colleagues [29] , in which furin initiates the reaction among precursors and results in covalently linked fluorescent oligomers inside cells. Although the increase of the local concentration of fluorescent gelators in the nanofibres of some organogels [39] , [40] results in improved contrast enhancement, we found that the choice of fluorophore is crucial because the replacement of NBD by rhodamine fails to provide the contrasts for imaging because the rhodamine derivative is a non-gelator. As many critical biological processes and targets are intracellular, the understanding of the evolution of the nanofibres inside cells promises the development of intracellular biomaterials that interact with biological entities. Moreover, because the fluorescence intensity correlates with the formation of the nanofibres inside cells, this molecule may serve as a model system in a phenotype assay to screen the inhibitors of fibrillar aggregates inside cells, which ultimately may provide leads for develop drugs for neurodegenerative diseases. Materials ALP was purchased from Biomatik USA, LLC., and NBD-Cl was purchased from TCI. General 1 and 2 were purified by a Waters Delta600 HPLC system equipped with an in-line diode array UV detector using a XTerra C18 RP column with CH 3 CN (0.1% of trifluoroacetic acid) and water (0.1% of trifluoroacetic acid) as the eluent. Liquid chromatography-mass spectrometry was obtained on Waters Acquity ultra Performance LC with Waters MICROMASS detector. NMR spectra were monitored on a Varian 400M NMR. Rheological test was performed on an ARES-G2 rheometer. TEM micrographs were obtained on a FEI Morgagni 268 electron microscope with a 1k CCD camera (GATAN, Inc., Pleasanton, CA, USA). Fluorescence spectra were measured on Shimadzu RF-5301-PC Fluorescence Spectrophotometer. Confocal images were obtained on a Leica TCS SP2 Spectral Confocal Microscope. Synthesis of compounds 1 was prepared by solid phase peptide synthesis using 2-chlorotrity resin and the corresponding Fmoc-protected amino acids. 1 H NMR (400 MHz, DMSO-d 6 ): δ 8.37 (d, 1H), δ 8.27 (d, 1H), δ 8.20 (m, 2H), δ 8.12 (d, 1H), δ 7.85–7.71 (m, 3H), δ 7.59 (s, 1H), δ 7.46 (m, 2H), δ 7.30–7.00 (m, 15H), δ 4.61–4.34 (m, 3H), δ 4.14 (m, 1H), δ 3.534 (q, 2H), δ 3.15–3.01 (m, 2H), δ 2.99–2.86 (m, 2H), δ 2.84–2.63 (m, 4H), δ 1.48–1.14 (m, 4H), δ 1.08–0.79 (m, 2H); 13 C NMR (100 MHz, DMSO-d 6 ): δ 172.7, 171.1, 171.0, 170.5, 169.8, 137.8, 137.7, 133.9, 132.9, 131.7, 129.7, 129.2, 129.1, 128.0, 127.9, 127.6, 127.4, 127.3, 127.2, 126.2, 126.1, 125.9, 125.4, 119.2, 119.1, 106.9, 61.7, 53.9, 53.6, 53.0, 52.9, 42.2, 37.5, 37.2, 35.5, 31.9, 26.6, 22.0; ESI MS ( m / z ): [M] + calcd. for C 45 H 50 N 5 O 10 P, 851.33; found [M+H] + , 852.49; found [M−H] − , 850.54. 2 : To a solution of 1 (50.0 mg, 58.7 μmol) and Na 2 CO 3 (12.4 mg, 117.4 μmol) in H 2 O was added NBD-Cl (58.7 μmol) dissolved in methanol. The mixture was stirred at 50 °C for 2 h, and then cooled to room temperature, neutralized with 10% HCl (aq). The solvent was removed under reduced pressure, and the crude product was purified by RP C18 HPLC (total yield: 67%). 1 H NMR (400 MHz, DMSO-d 6 ): δ 9.542 (s, 1H), δ 8.462 (d, 1H), δ 8.38–8.01 (m, 3H), δ 7.87–7.62 (m, 3H), δ 7.61–7.50 (d, 1H), δ 7.48–7.35 (m, 2H), δ 7.28–6.92 (m, 15 H), δ 6.35 (m, 2H), δ 4.69–4.12 (m, 4H), δ 3.54 (q, 2H), δ 3.07–2.63 (m, 8H), δ 1.79–1.18 (m, 6H); 13 C NMR (100 MHz, DMSO-d 6 ): δ 172.6, 171.4, 171.1, 170.6, 169.8, 137.7, 137.6, 133.8, 132.9, 131.7, 130.0, 129.2, 129.1, 128.0, 127.8, 127.6, 127.4, 127.3, 127.2, 126.2, 126.1, 125.9, 125.4, 119.7, 61.7, 53.8, 53.7, 52.2, 42.2, 37.5, 37.3, 35.9, 31.9, 27.3, 22.6, 20.8, 16.7; ESI MS ( m / z ): [M] + calcd. for C 51 H 51 N 8 O 13 P, 1014.33; found [M+H] + , 1015.4975; found [M−H] − , 1013.5474. Negative staining (I) Solutions and supplies: 2.0% (w/v) uranyl acetate (UA) (prepare by dissolving 200 mg UA in 10 ml of ddH 2 O. Add water to the tube containing UA, cover tube with foil and rotate in cold room for several hours till fully dissolved. Filter through a 0.22-μm filter that has be prerinsed well with ddH 2 O. Filtered stain stored at 4 °C in a foil-wrapped tube can be used for >1 year); filter strips (prepared by cutting Whatman 1 filter paper into small slivers); grids (400 mesh copper grids coated with continuous thick carbon film ~35 nm in thickness, purchased from Pacific Grid Tech. Co). (II) Negative staining protocol: (1) Glow discharge carbon-coated grids just before use to increase their hydrophilicity. (2) Place sample solution on the grid (3 μl, sufficient to cover the grid surface). (3) Rinsing: ~10 s later, place a large drop of the ddH 2 O on parafilm and let the grid touch the water drop, with the sample-loaded surface facing the parafilm. Tilt the grid and gently absorb water from the edge of the grid using a filter paper sliver three times. (4) (immediately after rinsing) Staining: place a large drop of the UA stain solution on parafilm and let the grid touch the stain solution drop, with the sample-loaded surface facing the parafilm. Tilt the grid and gently absorb the stain solution from the edge of the grid using a filter paper sliver three times. (5) Allow the grid to dry in air and examine the grid as soon as possible. Live cell imaging HeLa cells (CCL-2, 2×10 5 in 2 ml) were first placed in Glass Chamber (Thermo Scientific Nunc Lab-Tek, 2-well) and cultured in Eagle′s MEM (GIBCO) medium supplemented with 10% fetal bovine serum (FBS, GIBCO), 100 U ml −1 penicillin and 100 mg ml21 streptomycin (GIBCO) for 4 h to allow the cell attachment. Then the HeLa cells were washed three times with PBS buffer to replace the medium with PBS buffer. After the cell-containing glass chamber was fixed on the confocal microscope stage, the PBS buffer was replaced with 1 ml solution of 2 (500 or 50 μM dissolved in PBS buffer) and thereafter fluorescent images were captured immediately in the xyt mode with a delay of 11.64 s between frames. How to cite this article: Gao, Y. et al . Imaging enzyme-triggered self-assembly of small molecules inside live cells. Nat. Commun. 3:1033 doi: 10.1038/ncomms2040 (2012).